Structural snapshots of V/A-ATPase reveal the rotary catalytic mechanism of rotary ATPases V/A-ATPase is a motor protein that shares a common rotary catalytic mechanism with F o F 1 ATP synthase. When powered by ATP hydrolysis, the V 1 domain rotates the central rotor against the A 3 B 3 hexamer, composed of three catalytic AB dimers adopting different conformations (AB open , AB semi , and AB closed ). Here, we report the atomic models of 18 catalytic intermediates of the V 1 domain of V/A-ATPase under different reaction conditions, determined by single particle cryo-EM. The models reveal that the rotor does not rotate immediately after binding of ATP to the V 1 . Instead, three events proceed simultaneously with the 120˚ rotation of the shaft: hydrolysis of ATP in AB semi , zipper movement in AB open by the binding ATP, and unzipper movement in AB closed with release of both ADP and Pi . This indicates the unidirectional rotation of V/A-ATPase by a ratchet-like mechanism owing to ATP hydrolysis in AB semi , rather than the power stroke model proposed previously for F 1 -ATPase. The proton translocation ATPase/synthase family includes F-type enzymes found in eubacteria, mitochondria, and chloroplasts, and the V/A type enzymes found in archaea and some eubacteria [1] , [2] , [3] , [4] , [5] (Fig. 1A ). These ATPases produce the majority of cytosolic ATP from ADP and Pi using energy derived from the transmembrane proton motive force generated by cellular respiration [6] . These ATPases share a common molecular architecture, consisting of a hydrophilic V 1 /F 1 domain responsible for ATP hydrolysis or synthesis, and a hydrophobic V o /F o domain housing a proton translocation channel [7] , [8] , [9] . The chemical reaction (ATP hydrolysis/synthesis) in V 1 /F 1 is tightly associated with proton movement through V o /F o using a rotary catalytic mechanism, where both reactions are coupled by rotation of the central rotor complex relative to the surrounding stator apparatus, which includes the ATPase active hexamer [6] , [10] , [11] (Fig. 1B ). Fig. 1: Schematic representation of rotary ATPases and the conventional rotary mechanism. A Illustration of subunit composition of different types of rotary ATPases; prokaryotic V/A-ATPase ( left ), eukaryotic V-ATPase ( middle ), prokaryotic F-ATPase ( right ). The stators are represented in various colors and the rotors are represented in gray. B A schematic model of the rotary catalytic mechanism of the V/A-ATPase. When powered by ATP, the central rotor composed of D 1 F 1 d 1 c 10 (gray) rotates against a surrounding stator composed of A 3 B 3 E 2 G 2 a 1 (white), coupled with proton translocation across the membrane. C The conventional catalytic cycle of V/A-ATPase. At low ATP concentration, the ATP binding dwell time is increased. ATPγS also prolongs the ATP hydrolysis dwell. Full size image The V/A-ATPase from the thermophilic bacterium, Thermus thermophilus ( Tth ) is one of the best-characterized ATP synthases [3] , [12] . The overall architecture and subunit composition of V/A-ATPase is more similar to that of the eukaryotic V-ATPase, rather than F-type ATPase. However, the Tth V/A-ATPase has a simpler subunit structure than the eukaryotic V-ATPase and shares the ATP synthase function of F-type ATPase [13] (Fig. 1A ). The V 1 domain of Tth V/A-ATPase (A 3 B 3 D 1 F 1 ) is an ATP-driven rotary motor where the central DF shaft rotates inside the hexameric A 3 B 3 containing three catalytic sites, each composed of an AB dimer. The V o domain (E 2 G 2 d 1 a 1 c 12 ) is composed of stator parts including the a subunit and two EG peripheral stalks and the d 1 c 12 rotor complex, which consists of a central rotor complex with the DF subunits of V 1 [14] , [15] , [16] . When ATP hydrolysis by A 3 B 3 powers the DF shaft, the reverse rotation of the central rotor complex drives proton translocation in the membrane-embedded V o domain (Fig. 1B ). According to the binding change mechanism of ATP synthesis [6] , the three catalytic sites in ATP synthases are in different conformations but interconvert sequentially between three different conformations as catalysis proceeds. Indeed, our previous structure demonstrated that the A 3 B 3 hexamer in the V/A-ATPase adopts an asymmetrical structure composed of three different AB dimers, termed open (AB open ), semi-closed (AB semi ), and closed (AB closed ) [16] , [17] . Experimental studies using specific rotational probes attached to DF revealed that ATP-driven rotation of the central shaft was unidirectionally clockwise when viewed from the V 1 side [10] . At low ATP concentrations where ATP binding is rate-limiting, rotation proceeds in steps of 120°, commensurate with the three catalytic sites of AB dimers [18] . When using 40 nm gold beads with almost negligible viscous resistance, V 1 also pauses every 120° even at an ATP concentration around K m without a sign of substeps [19] . These single-molecule experiments on V 1 suggest that both catalytic events, ATP hydrolysis and product (ADP and Pi ) release occur at an individual ATP binding position, and imply the presence of chemo-mechanically stable catalytic intermediates (Fig. 1C and Supplementary Fig. 1 ). However, single-molecule observation experiments only allow us to see the motion of the shaft to which the observation probe is bound, and do not tell us what events are occurring at each catalytic site. To elucidate the entire rotational mechanism of the V/A-ATPase, we must determine the structures of catalytic intermediates of the rotary ATPase during rotation. There are many reaction intermediates of the enzyme during turnover, and this structural heterogeneity makes successful crystallization of a specific state very challenging. Technological breakthroughs in single-particle Cryo-EM, such as the development of direct electron detectors, and advances in image processing and automation [20] , [21] , have triggered a revolution in structural biology, making this the technique of choice for large and dynamic complexes unsuitable for crystallization. In addition, by freezing Cryo-EM grids at different time points or under different reaction conditions, it is possible to trap intermediate states and thus build up a picture of the chemo-mechanical cycle of biological macromolecular complexes step by step. To date, there are few examples of studies that have successfully captured such details of a catalytic cycle at atomic resolution using Cryo-EM [22] , [23] . Here, we report several keys, and thus far uncharacterized, intermediate states of V/A-ATPase, obtained under different reaction conditions. Comparison of these structures provides insight into the cooperativity between the three catalytic sites and demonstrates a rotary catalytic mechanism powered by ATP hydrolysis. Sample preparation for Cryo-EM structural analysis We previously determined the Cryo-EM structures of the wild-type V/A-ATPase containing an ADP in the catalytic site of AB closed [16] , [17] . The V/A-ATPase bound to the inhibitory ADP exhibits no ATPase activity until the ADP is removed [13] , [16] , [24] . 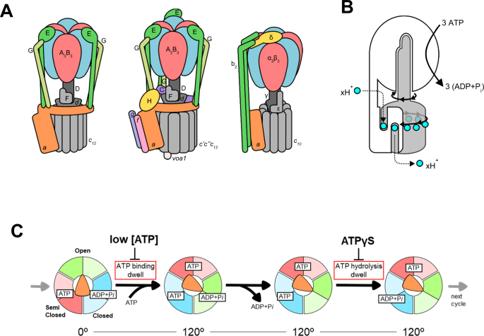Fig. 1: Schematic representation of rotary ATPases and the conventional rotary mechanism. AIllustration of subunit composition of different types of rotary ATPases; prokaryotic V/A-ATPase (left), eukaryotic V-ATPase (middle), prokaryotic F-ATPase (right). The stators are represented in various colors and the rotors are represented in gray.BA schematic model of the rotary catalytic mechanism of the V/A-ATPase. When powered by ATP, the central rotor composed of D1F1d1c10(gray) rotates against a surrounding stator composed of A3B3E2G2a1(white), coupled with proton translocation across the membrane.CThe conventional catalytic cycle of V/A-ATPase. At low ATP concentration, the ATP binding dwell time is increased. ATPγS also prolongs the ATP hydrolysis dwell. Partial ADP removal from AB closed is possible by dialysis against an EDTA-phosphate buffer, but it is difficult to obtain a homogenous nucleotide-free V/A-ATPase after such a treatment, due to the high binding affinity of the ADP to AB closed (Supplementary Table 1 ). To obtain a homogeneous ATPase active enzyme, mutant V/A-ATPase (A/S232A, T235S) with reduced nucleotide-binding affinity was purified from T. thermophilus membranes [10] . The mutated V/A-ATPase exhibits higher K m values for nucleotide in both the ATP hydrolysis and synthesis reactions than the wild-type enzyme, but the enzymatic and rotational properties are almost the same as those of the wild-type enzyme [24] . The mutated V/A-ATPase is fully activated for ATPase activity after EDTA/phosphate dialysis; no ADP or ATP was found in the enzyme by quantitative analysis of nucleotides (Supplementary Fig. 2 and Table 1 ). We incorporated the nucleotide-free V/A-ATPase into nanodiscs comprising the MSP1E3D1 scaffold protein and DMPC. The resulting V/A-ATPase obeys simple Michaelis–Menten kinetics and exhibits ATPase activity of 22 s −1 and the K m of 394 µM ATP (Supplementary Fig. 2b ). The nucleotide-free V/A-ATPase (Nucfree) was used for cryo-grid preparation under different ATPase reaction conditions (Supplementary Fig. 1c ). Results of the structural analysis of the protein under each set of reaction conditions are summarized in Supplementary Fig. 3a–d . The structures of V/A-ATPase without nucleotide (V nucfree ) The flow charts showing image acquisition and reconstitution of the 3D structure of V/A-ATPase without nucleotide are summarized in Supplementary Fig. 3a . We obtained structures of three rotational states of V/A-ATPase without nucleotide; state1 at 3.1 Å, state 2 at 4.7 Å, and state 3 at 6.3 Å resolution, with the DF shaft positions differing by 120° in each case (Fig. 2 ). Using signal subtraction of the V o domain, we achieved resolution of 3.0 and 4.1 Å for the V 1 domain including half of the EG stalk in state1 and 2, allowing us to build atomic models of the V 1 domain of these states. Fig. 2: Cryo-EM density map and the atomic model for nucleotide-free V/A-ATPase. A Cryo-EM density map of whole V/A-ATPase of state1 in the absence of nucleotide (V nucfree structure). B Cryo-EM density map of V 1 EG of state1 without nucleotide ( left ). Cross-sections of the nucleotide-binding sites ( right upper ) and A 3 B 3 C-terminal region ( right lower ) viewed from the top. C Comparison of the AB dimer structures in V nucfree . AB dimers are shown as space-filling models and superimposed on the β barrel domain (A subunit 1–70 a.a.). Left; AB open (solid) vs. AB semi (semi-transparent), middle; AB open (solid) vs. AB closed (semi-transparent), and AB semi (solid) vs. AB closed (semi-transparent). D Comparison between each AB subunit in V nucfree . The subunits are shown as wire representations. A and B subunits are superimposed on the β barrel domain. Full size image The three AB dimers in the V 1 domain adopted open (AB open ), semi-closed (AB semi ), and closed (AB closed ) states, respectively (Fig. 2 B, C). The tip of the C-terminal helix bundle (CHB) of A open is in contact with the C-terminal helix of the D subunit, and the wide part of the CHB of B open is in contact with the N-terminal helix of the D subunit, respectively (Supplementary Fig. 4a–c ). The AB semi and AB closed also interact with the coiled-coil of subunit D in specific regions of the CHB, respectively (Supplementary Fig. 4d–g ). The differences in the structures of the three AB dimers, when superimposed on the β barrel domains of both A and B subunits, are the result of the movement of the N-terminal bulge domain, the nucleotide-binding domain (NB) of the A subunit and the CHBs of both the A and B subunits (Fig. 2D ). When comparing the structure of AB open and AB semi , both the NB and CHB of the A semi are in closer proximity to B semi than B open , resulting in a closed structure of AB semi (Fig. 2C , D). The structure of B open is very similar to B semi , as shown in Fig. 2D . In the AB closed , both the CHB and NB domains of A closed are in closer proximity to B closed , and the CHB of B closed moves to A closed , resulting in the more closed structure of AB closed compared to AB semi (Fig. 2C, D ). In the AB closed and AB semi dimers, densities for the catalytic side chains are well resolved, but no density corresponding to nucleotide was observed (Fig. 3A ). Hereafter we refer to the structure as the V nucfree . The structure of V nucfree is very similar to the previously reported ADP inhibited structure [16] , [17] . For state1, the rmsd value for the C α chains of A 3 B 3 DF of the V nucfree and ADP inhibited structures is 1.98 Å (Supplementary Fig. 5 ). In addition, the V nucfree is also similar to the structures under the saturated-ATP condition determined in this study, with the positions of the catalytic side chains almost identical in both cases (Supplementary Fig. 6 ). This indicates that the V 1 domain adopts the same conformation, including the arrangement of the DF shaft in the A 3 B 3 and the geometry of the catalytic side chains, irrespective of the presence or absence of bound ATP. Fig. 3: Structures of nucleotide-binding sites obtained in each condition. Upper panels: V nucfree ( A ), V prehyd ( B ), V 3nuc ( C ), and V 2nuc ( D ) viewed from the cytosolic side. The scale bar is 20 Å. Magnified views of the three nucleotide-binding sites (AB open , AB semi , and AB closed ) in each structure are shown in the rows below. Cryo-EM maps are represented as semi-translucent. Bound nucleotides and Mg ions are shown in ball-and-stick and sphere representation, respectively. The scale bar is 4 Å. Full size image In the density maps obtained for state1 of V nucfree , the CHB of the AB dimers was slightly blurred, likely due to structural heterogeneity. To classify the probable substates of state1, we performed focused 3D classification using a mask covering AB open and B semi (Supplementary Fig. 3a ). We identified a cryoEM structure of the original state1 from 39,902 particles at 3.1 Å resolution and another substate from 24,101 particles at 3.1 Å resolution. We termed the substates reconstructed from these major particle classes as state1-1 and state1–2, respectively. The atomic model initially constructed as state1 is identical to the atomic model of state1–1. The structures of the sub-states are very similar, with most differences due to the movement of the CHB of the A and B subunits. Therefore, we quantified the difference in the structure of the CHB observed when the structures were superimposed on the N-barrel domain (Supplementary Tables 2 and 3 ). Substates were also obtained under other reaction conditions (see below) and the rmsd values shown in Supplementary Tables 2 and 3 are used to discuss which subunits are responsible for the differences in the structure of the substates obtained under different reaction conditions. Structures obtained at a saturating ATP concentration Cryo-grids were prepared using a reaction mixture of nucleotide-free V/A-ATPase, containing the regenerating system and ATP at a saturating concentration of 6 mM. The reaction mixture was incubated for 120 s at 25 °C and then loaded onto a holey grid, followed by flash freezing. We determined three rotational states followed by focused refinement using a V 1 EG mask for each state (Supplementary Fig. 3b ). In the density maps obtained for each state, the amino acid residues of the nucleotide-binding sites in both AB closed and AB semi were well resolved, but the CHB domains of the AB dimers were blurred due to structural heterogeneity, as with the V nucfree . For state1, we identified an atomic resolution structure of state1-1 from 40,831 particles at 3.1 Å resolution and state1–2 from 28,801 particles at 3.2 Å resolution by further 3D classification without alignment (Supplementary Fig. 3b ). The same classification analysis was performed for state2 and state3, yielding state 2–1 (3.0 Å resolution) and state 2–2 (3.4 Å resolution), and state 3–1 (3.0 Å resolution) and state 3–2 (3.4 Å resolution) respectively. In these structures, nucleotide densities have been identified in the three catalytic sites. Hereafter, we refer to the structures obtained at ATP saturating conditions as V 3nuc . The structure of AB open of V 3nuc state1–1 is almost identical to that of V nucfree state1–1 (Supplementary Fig. 6 ). This is confirmed by the fact that the rmsd values in the CHB of A open and B open for V 3nuc state1–1 and V nucfree are less than 1 Å (Supplementary Tables 2 and 3 ). The AB open of state1–2 adopts a slightly more closed conformation compared to that of state1–1, which results from a movement of CHB of B open toward the β-barrel domain (Fig. 4C ). Nevertheless, the AB open of V 3nuc with bound ATP retains the interaction with the DF shaft, indicating that ATP binding to the AB open does not move the DF shaft. Fig. 4: Comparison between state1–1 and 1–2 in each subunit of V 3nuc . The subunits of state1–1 and 1–2 were superimposed on the β barrel domain (A: 1–70 a.a., B: 1–70 a.a.). Ribbon models are colored by the rmsd values calculated for the atoms of the main chain; gray (small changes) to red (large changes). 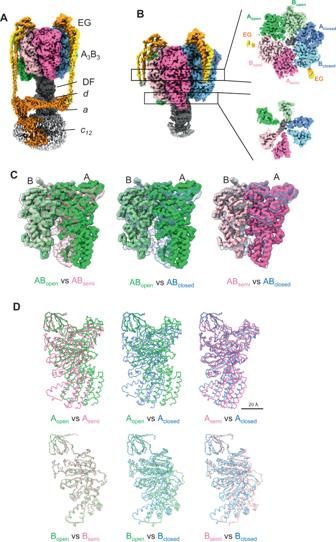Fig. 2: Cryo-EM density map and the atomic model for nucleotide-free V/A-ATPase. ACryo-EM density map of whole V/A-ATPase of state1 in the absence of nucleotide (Vnucfreestructure).BCryo-EM density map of V1EG of state1 without nucleotide (left). Cross-sections of the nucleotide-binding sites (right upper) and A3B3C-terminal region (right lower) viewed from the top.CComparison of the AB dimer structures in Vnucfree. AB dimers are shown as space-filling models and superimposed on the β barrel domain (A subunit 1–70 a.a.).Left;ABopen(solid) vs. ABsemi(semi-transparent),middle;ABopen(solid) vs. ABclosed(semi-transparent), and ABsemi(solid) vs. ABclosed(semi-transparent).DComparison between each AB subunit in Vnucfree. The subunits are shown as wire representations. A and B subunits are superimposed on the β barrel domain. Magnified views of the CHBs are represented in the lower panels as wire models. The models of state1–1 are represented in gray, and state1–2 are represented in different colors. A Subunits in AB closed , B subunits in AB semi , C subunits in AB open . Full size image The AB semi in state1–2 has a more closed structure than that in state1–1 mainly due to the movement of CHB in B semi (Fig. 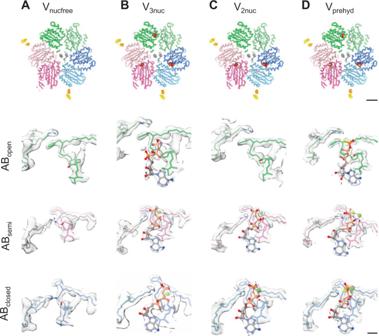Fig. 3: Structures of nucleotide-binding sites obtained in each condition. Upper panels:Vnucfree(A), Vprehyd(B), V3nuc(C), and V2nuc(D) viewed from the cytosolic side. The scale bar is 20 Å. Magnified views of the three nucleotide-binding sites (ABopen, ABsemi, and ABclosed) in each structure are shown in the rows below. Cryo-EM maps are represented as semi-translucent. Bound nucleotides and Mg ions are shown in ball-and-stick and sphere representation, respectively. The scale bar is 4 Å. 4B , Supplementary Table 3 ). In summary, V 3nuc state1–2 has a more closed structure than state1–1 due to the movement of the CHB of both A semi and B semi , but the slightly closed conformation of state1–2 is independent of ATP binding to the AB open . Structures of the catalytic sites at AB dimers of V 3nuc In both state1–1 and state1–2 structures obtained under ATP saturating conditions, a bound ATP molecule is clearly observed in the catalytic site of AB open (Fig. 3B and Supplementary Fig. 7c ). The catalytic sites in the AB closed and AB semi in both the state1–1 and state1–2 also contained density corresponding to an ATP molecule, and in these cases, the associated magnesium ions were visible (Fig. 3B and Supplementary Fig. 7a, b ). In the V 3nuc structure, we did not find density corresponding to nucleotides between the D and A subunits as reported in a previous paper [25] (Supplementary Fig. 8 ). In the catalytic site of AB semi of V 3nuc , the density of each nucleotide phosphate atom was easily identifiable (Supplementary Fig. 7b ), indicating that the ATP molecule occupies the catalytic site in AB semi . The protein structure is sufficiently clear to also provide a detailed picture of the configuration of the catalytic side chains (Fig. 5A–C ). The γ-phosphate of ATP and the magnesium ion are coordinated by the A/K234 and A/S235 residues on the P-loop, which contains the conserved nucleotide-binding motif [26] . The aromatic ring of A/F230, not conserved in F type ATPase, is oriented away from the triphosphate moiety, allowing access of the guanidium group to the arginine finger (Supplementary Fig. 9 ). Considering clear EM density for the γ-phosphate of the ATP bound in AB semi , hydrolysis of ATP is unlikely to proceed in AB semi . Fig. 5: Coordination of nucleotides in the binding sites of V 3nuc and V prehyd . Left panels; Comparison of the three nucleotide-binding sites (AB open ( A ), AB semi ( B ), and AB closed ( C )) of state1–1 of V 3nuc shown with colored (green, blue, and pink) atoms and bonds, and main chain, and state1–1 of V prehyd shown with gray atoms, bonds and main chain. Right panels; schematic representations of the coordination of the ATP group in the three binding sites of V 3nuc and V prehyd in parentheses. The distances between the atoms are shown in dotted lines. All distances are in Å. Full size image The nucleotide-binding site of the AB closed is shown in Fig. 5B . The geometry of ATP binding in AB closed is very similar to that found in the AB semi , however, the carbonyl group of A/E257 is closer to the γ-phosphate by about 1 Å than AB semi . In state1–2 of V 3nuc , the γ-phosphate of ATP bound to the AB closed appears to be separated from β-phosphate when a relatively high density threshold is used (Supplementary Fig. 10 ). These findings strongly suggest that ATP bound to AB closed is either already hydrolyzed or in the process of being hydrolyzed. The state of ATP in AB closed is discussed further in Supplementary Note . In the nucleotide-binding site of the AB open of V 3nuc , the adenosine moiety of ATP is occluded as in the AB semi and AB closed , with A/F415, A/Y500, and A/V236 forming the adenine binding pocket, however, the hydrogen bonding of the ribose moiety to the side chain of B/N363 is lost due to movement of the CHB of A open (Fig. 5C ). Unlike in the AB closed and AB semi , the phenyl group of A/230F in the AB open is closer to the tri-phosphate group of ATP due to the torsion of the main chain, resulting in the formation of a hydrophobic barrier between the catalytic side chains and the triphosphate moiety of ATP (Supplementary Fig. 9 ). Compared with AB semi , the side chains of catalytic residues A/E257, A/R258, and B/R360 of AB open are much further away from the γ-phosphate of ATP (10.0, 10.0, and 7.1 Å, respectively. Consequently, the configuration of the catalytic residues in the nucleotide-binding site of AB open is not appropriate for hydrolysis of the bound ATP. Instead, the bound ATP has the potential to zipper the AB interface via interaction with the surrounding catalytic residues, which ultimately results in the transition of AB open to a more closed form via a typical zipper conformational change. Structures of V/A-ATPase waiting for ATP to bind To determine the ATP-waiting structure of V/A-ATPase, we prepared a cryo-grid with a reaction mixture containing 4 µM enzyme, 50 µM ATP, and the ATP regeneration system, pre-incubated for 300 s. We reconstructed three rotational states (state1, 2.7 Å, state2, 3.3 Å, and state3 3.6 Å resolution) from the single-particle images of the holo-complex and three rotational states of V 1 EG (state1, 2.8 Å, state2, 3.1 Å, and state3, 2.8 Å) by focused masked refinement. For state1, two substates (state1–1, 2.9 Å and state1–2, 3.0 Å) were separated by focused classification using AB open and AB semi masks (Supplementary Fig. 3c ). In both AB semi and AB closed of state1–1, the apparent density of ATP-magnesium was observed, but the density of the γ-phosphate at the AB closed is weaker than that at the AB semi (Fig. 3C and Supplementary Fig. 7a, b ). In contrast, density was not observed in the nucleotide-binding site of AB open . For state1–2, as in state1–1, nucleotides are present in both AB semi and AB closed , while AB open is empty. Hereafter we refer to the structure as V 2nuc . The overall structure and geometry of the catalytic residues of state1–1 of V 2nuc are largely identical to state1–1 of V nucfree and V 3nuc (Supplementary Fig. 11 ). This structural similarity between V 2nuc , V nucfree , and V 3nuc is confirmed by the low rmsd values when comparing the CHB of the A and B subunits of these structures (Supplementary Tables 2 and 3 ). The similarity of the structures of these substrates indicates that the structural polymorphism of the V 1 domain is independent of the binding of ATP to AB dimers. Structures obtained at a saturating concentration of ATPγS (V prehyd ) The V 1 -ATPase from T. thermophilus is capable of hydrolyzing ATPγS, however, the turnover rate of ATPγS is much lower than that of ATP due to the decrease in hydrolysis rate [18] (Supplementary Fig. 2d ). Thus, pre-hydrolysis structures of V/A-ATPase can be obtained at 4 mM ATPγS. The cryo-grid was prepared by blotting of the reaction mixture comprising Nucleotide-free V/A-ATPase and 4 mM of ATPγS in the absence of the regenerating system in order to exclude any effect of regenerated ATP produced from hydrolyzed ATPγS. We reconstructed three rotational states from the acquired EM images using the CRYOARM300 (JEOL). After the focused masked refinement of the V 1 EG domain, we obtained atomic resolution structures of each state (state1, 2.7 Å, state2, 3.4 Å, and state3, 3.6 Å), respectively (Supplementary Fig. 3d ). We refer to these structures as V prehyd . For state1, two sub-states, state1–1 and state1–2, were obtained at 2.7 and 2.9 Å resolution respectively, by focused classification using a mask with AB open and AB semi (Supplementary Fig. 3d ). For the AB open of V prehyd , bound ATPγS is clearly observed in the catalytic site, which has an almost identical structure to that of the ATP bound state of V 3nuc (Fig. 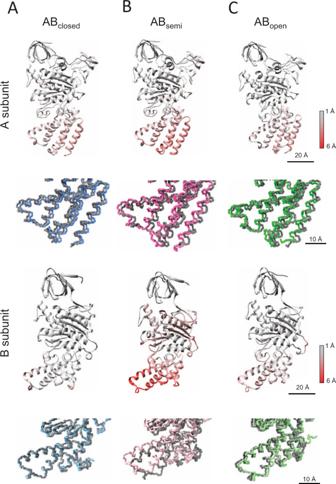Fig. 4: Comparison between state1–1 and 1–2 in each subunit of V3nuc. The subunits of state1–1 and 1–2 were superimposed on the β barrel domain (A: 1–70 a.a., B: 1–70 a.a.). Ribbon models are colored by thermsdvalues calculated for the atoms of the main chain; gray (small changes) to red (large changes). Magnified views of the CHBs are represented in the lower panels as wire models. The models of state1–1 are represented in gray, and state1–2 are represented in different colors.ASubunits in ABclosed,Bsubunits in ABsemi,Csubunits in ABopen. 3B ). The nucleotide-binding sites of the AB closed and AB semi of V prehyd are almost identical to those of V 3nuc , respectively, as shown in Fig. 5 . The γ-phosphate group of the bound ATPγS molecule in the AB semi is well resolved as seen in for ATP in V 3nuc and V 2nuc (Fig. 3d and Supplementary Fig. 7b ). In contrast, the density of γ-phosphate of ATPγS at the AB closed is faint (Supplementary Fig. 7a ), suggesting that the ATPγS in the AB closed has already been hydrolyzed and the bound nucleotide in the AB closed is ADP. This indicates that the AB semi is in the pre-hydrolysis conformation, waiting for ATP hydrolysis. We have obtained catalytic intermediates of the V 1 domain, V nucfree , V 3nuc , V 2nuc , and V prehyd , with different nucleotide occupancy. Despite the different nucleotide occupancy of these structures, their overall conformations are very similar. For instance, the rmsd of the C α chains of A 3 B 3 in V nucfree and V 3nuc state1–1 is 1.98 Å. In addition, the relative position of the central DF shaft within the asymmetric A 3 B 3 is almost the same in the V nucfree and V 3nuc structures. These findings demonstrate that the configuration between the DF shaft and individual AB dimers is independent of the state of nucleotide occupancy of each AB dimer. In other words, the structure of the V 1 domain adopts three rotational states, 1–3, during continuous ATP hydrolysis, with the conformational changes in the A 3 B 3 hexamer driven by ATP hydrolysis, being discrete rather than continuous. The V 3nuc structure, obtained under ATP saturation conditions shows all three catalytic sites occupied by ATP or the products of hydrolysis (ADP + Pi ). Since the hydrolyzed Pi is clearly visible in the AB closed of V 3nuc (Supplementary Fig. 10 ), it is assumed that V 3nuc is the structure before dissociation of Pi from the catalytic site in AB closed . We also obtained the V 2nuc structure in which ATP and product(s) are bound to AB semi and AB closed , respectively, but AB open is empty. The V 2nuc is therefore assumed to be the structure of the protein awaiting ATP binding to AB open . When using ATPγS as a substrate, which has a very slow hydrolysis rate, the high-resolution atomic structure of the V 1 domain allowed visualization of ATPγS molecules bound to the catalytic sites of AB open and AB semi , as well as identification of the hydrolyzed ATPγS at the AB closed . The V prehyd reveals both that the AB closed adopts the post-hydrolysis state where the product of phosphate ( Pi ) is dissociated, and that the AB semi is awaiting ATP hydrolysis. The structures provide important insights into the chemo-mechanical cycle of V/A-ATPase. The V/A-ATPase undergoes a unidirectional conformational change from state1 to state2 to state3 when powered by ATP. Thus, V 3nuc of state1, in which three catalytic sites are already occupied by nucleotides, should change to state2 of V 2nuc , following ATP hydrolysis at AB semi , and the subsequent or simultaneously dissociation of ADP and Pi by the discrete structural transition of AB closed to AB open (Fig. 6 ). This demonstrates that rotation of the rotary ATPase proceeds via the tri-site model with the protein progressing through a two nucleotide bound state and a three-nucleotide bound state, settling the long-standing debate on whether the bi-site model or tri-site model is appropriate for rotary ATPases [5] , [6] , [27] , [28] , [29] , [30] . Fig. 6: Chemo-Mechanical cycle of V/A-ATPase driven by ATP hydrolysis. The structures of V/A-ATPase viewed from the cytosolic side are shown as ribbon models. The coiled-coil of the DF subunits is shown in gray. The bound ATP molecules are highlighted in sphere representations. State1–1 and 1–2 of V 2nuc are in equilibrium and are fluctuating. These structures transit to state1–1 and 1–2 of V 3nuc by ATP binding to AB open , without a 120° rotation step of the DF rotor. V 3nuc in state1–1 and state1–2 are also in equilibrium. ATP hydrolysis at AB semi and zipper motion at AB open occur simultaneously. This triggers the transition of V 3nuc in state1–2 to V 2nuc state2–2 together with the 120° rotation step and simultaneous release of ADP and Pi . State2 of V 2nuc returns to state1 via state3 of V 2nuc by the same process. Asterisks indicate the structures which were not identified in this study. Full size image Based on previous single molecular observation experiments for both F 1 - and V 1 -ATPase, ATP binding onto the enzyme directly triggers the first 120° rotation step of the DF shaft [18] , [19] , [30] (Supplementary Fig. 1a ). In light of our findings presented here, this scheme needs to be redrawn; the rotor does not immediately travel 120° as a result of ATP binding to enzyme. The next catalytic event after ATP binding is ATP hydrolysis in AB semi . Each conformational change, from AB open to AB semi , AB semi to AB closed , and AB closed to AB open occurs simultaneously, with the rotation of the shaft, and with the hydrolysis of ATP in the AB semi and release of products (ADP and Pi ) from the AB closed (Fig. 6 and Supplementary Movie 1 ). This is in contrast to the classical rotary model, where catalytic events occur in sequence at the three catalytic sites, until now the broadly accepted mechanism of action of the F 1 -ATPase [6] , [27] , [31] , [32] . In the V 2nuc and V 3nuc , two sub-states, state1–1 and state1–2 were identified (Supplementary Fig. 12 ). These substrates were also identified in V nucfree , thus the conformational dynamics of the V 1 domain are independent of ATP binding. In other words, state1–1 and state1–2 are in a thermal equilibrium state, irrespective of nucleotide occupancy in each catalytic site. Both AB semi and AB open in state1–2 adopt more closed structures than those in state1–1, suggesting that state1–2 of V 3nuc is likely an intermediate structure just prior to the 120° rotation step of the DF shaft. Compared to state1–2 of V 3nuc , state1–2 of V prehyd exhibits slightly more closed structures of AB open and AB semi (Supplementary Fig. 13 ), likely to be associated with the progress of the catalytic reaction in AB closed , i.e., the dissociation of the phosphate. In this respect, state1–2 of V prehyd may be another reaction intermediate structure in which the Pi in the AB closed is released prior to the 120° step (Supplementary Fig. 14 ). Based on the catalytic intermediates of the V 1 domain of V/A-ATPases obtained under four different reaction conditions, we propose a model for the ATP-driven rotation mechanism of V/A-ATPases (Fig. 7 , Supplementary Fig. 15 ). Fig. 7: The rotary mechanism of V/A-ATPase powered by ATP hydrolysis. The schematic models of AB open , AB semi , and AB closed are shown in green, pink, and blue, respectively. The coiled-coil region of the D subunit in contact with A 3 B 3 is shown in gray. In the ADP inhibited state, the entrapped ADP in AB closed hampers the structural transition of AB open to AB semi by binding of ATP to AB open . The V nucfree in the ground state is activated by the binding of ATP to the catalytic sites. In V 2nuc awaiting ATP binding, binding of ATP to AB open does not induce the 120° rotation step. In V 3nuc , both zipper motion of AB open and ATP hydrolysis in AB semi induce unzipper motion of AB closed accompanying the release of ADP and Pi . The catalytic events in the three AB dimers occur simultaneously with the 120˚ step of the DF shaft, resulting in the structural transition of state1 of V 3nuc to state2 of V 2nuc . Full size image When ATP binds to V nucfree , which is in a stable initial state (ground state), the enzyme transits into the steady-state for ATP hydrolysis (Fig. 7 , upper row ). The V 3nuc structure is formed by binding of ATP to the AB open of V 2nuc but the binding of ATP itself does not cause structural transitions between AB dimers associated with the 120° step of the DF shaft. In the V 3nuc structure, where nucleotides are bound to all three AB dimers, three distinct but associated catalytic events occur at the three AB dimers simultaneously and these events are coupled to the first 120° rotation step of the DF shaft. One of the driving events for this transition is the conformational change from the ATP-bound AB open to the more closed AB semi , which can be explained by a zipper motion of AB open occurring upon ATP binding. From our structures, a comparison between AB open and AB semi implies that new hydrogen bonds form between the triphosphate moiety of ATP and the surrounding side chain groups of B/R360, A/258R, A/257E, and A/K234 (Fig. 5 ). The V prehyd structures indicate that the ATP bound to AB semi is awaiting hydrolysis. The conformational change from AB semi to AB closed should occur spontaneously because it involves ATP hydrolysis, an exergonic reaction. In contrast, ADP bound to AB closed hampers the unzipper motion in AB closed , thereby preventing the overall structural transition of the V 1 domain. This is supported by the fact that V/A-ATPase adopts the ADP inhibited state in which ADP is entrapped in AB closed (Fig. 7 , upper line). The enzyme in the ADP-inhibited state does not show ATP hydrolysis activity even at saturated ATP concentration [13] , [16] . In summary, the ATP-driven unidirectional rotation of V/A-ATPase proceeds by a discrete structural transition between the three rotational states, i.e., the potential barrier to the structural transition of AB closed to AB open , accompanied by the release of ADP and Pi , is overcome by both a zipper motion of AB open by the bound ATP and ATP hydrolysis in AB semi . Since the ATP hydrolysis reaction is a heat dissipation process, the structural transition of AB semi to AB closed associated with the ATP hydrolysis occurs spontaneously and irreversibly, resulting in a unidirectionality of the 120° steps of the rotor. In other words, our model explains the unidirectional rotation by a ratchet-like mechanism driven by ATP hydrolysis, rather than the power stroke model proposed previously for F 1 -ATPase [5] , [33] . V/A-ATPase and F o F 1 are molecular machines based on the same construction principle, and thus are likely to share the same rotary mechanism. In fact, observation of rotation with high time-resolved rotation analysis using a tiny gold rod showed that bacterial F-ATPase and an A-ATPase share the same rotation mechanism [34] . For both rotary ATPases, a 120° rotation step together with ATP hydrolysis occurs after the catalytic dwell under ATP-saturated conditions. Importantly, for the thermophilic F 1 , the first 120° rotation step also includes ~80° and ~40° substeps, suggesting the existence of at least one additional catalytic intermediate of F 1 [5] , [27] , [35] . A recent structural study of thermophilic F 1 -ATPase indicated a possible intermediate structure responsible for the substeps [32] . In the V/A-ATPase, any intermediate structure containing phosphate after ADP or Pi release is likely to be in an unstable state, and therefore studies on the ATP-driven rotation of V/A-ATPase have failed to reveal the presence of any substep [19] . Preparation of Tth V/A-ATPase for biochemical assay and cryo-EM imaging The Tth V/A-ATPase containing His3 tags on the C-terminus of each c subunit and the TSSA mutation (S232A and T235S) on the A subunit was isolated from T. thermophilus membranes as previously described [24] with the following modifications. The enzyme, solubilized from the membranes with 10% Triton X-100 was purified by Ni 2+ -NTA affinity with 0.03% dodecyl-β- d -maltoside (DDM). For bound nucleotide removal, the eluted fractions containing Tth V/A-ATPase were dialyzed against 200 mM Sodium phosphate, pH 8.0, 10 mM EDTA, and 0.03% DDM overnight at 25 °C with three buffer changes, followed by dialysis against 20 mM Tris-Cl, pH 8.0, 1 mM EDTA, and 0.03% DDM (TE buffer) prior to anion exchange chromatography using a 6 ml Resource Q column (GE healthcare). The Tth V/A-ATPase was eluted by a linear NaCl gradient using a TE buffer (0–500 mM NaCl, 0.03% DDM). The eluted fractions containing holo - Tth V/A-ATPase were concentrated to ~10 mg/ml using Amicon 100k molecular weight cut-off filters (Millipore). For nanodisc incorporation, the 1,2-Dimyristoyl-sn-glycero-3-phosphorylcholine (DMPC, Avanti) was used to form lipid bilayers in reconstruction as previously described [16] . Purified Tth V/A-ATPase solubilized in 0.03% n-DDM was mixed with the lipid stock and membrane scaffold protein MSP1E3D1 (Sigma) at a specific molar ratio V o V 1 :MSP:DMPC lipid = 1:4:520 and incubated on ice for 0.5 h. Then, 200 μL of Bio Beads SM-2 equilibrated with a wash buffer (20 mM Tris-HCl, pH8.0, 150 mM NaCl) was added to the 500 μL mixture. After 2 h incubation at 4 °C with gentle stirring, an additional 300 μL of Bio Beads was added and the mixture was incubated overnight at 4 °C to form the nanodiscs. The supernatant of the mixture containing nanodisc- Tth V/A-ATPase (nd-V/A-ATPase) was loaded onto the Superdex 200 Increase 10/300 column equilibrated with wash buffer. The peak fractions were collected, analyzed by SDS-PAGE, and concentrated to ~4 mg/mL. The prepared nd -V/A-ATPase was immediately used for biochemical assay or cryo-grid preparation since nd -V/A-ATPase aggregates within a few days. Biochemical assay The quantitative analysis of bound nucleotides of Tth V/A-ATPase was carried out using anion-exchange high-performance liquid chromatography [13] . Bound nucleotides were released from the enzyme by the addition of 5 μl of 60% perchloric acid to 50 μl of the enzyme solution. Thereafter, the mixture was incubated on ice for 10 min. Then, 5 μl of 5 M K 2 CO 3 solution was added and the mixture was incubated on ice for 10 min. The resulting pellet was removed by centrifugation at 4 °C. The supernatant was applied to a Cosmopak-200 column equilibrated with 0.1 M sodium phosphate buffer (pH 7.0). The column was eluted isocratically with the same buffer at a flow rate of 0.8 ml/min. The nucleotide was monitored at 258 nm. The peak area was determined by automatic integration. ATPase activity was measured at 25 °C with an enzyme-coupled ATP-regenerating system, as described previously [13] . The reaction mixture contained 50 mM Tris-HCl (pH 8.0), 100 mM KCl, different concentrations of ATP-Mg, 2.5 mM phosphoenolpyruvate (PEP), 50 μg/ml pyruvate kinase (PK), 50 μg/ml lactate dehydrogenase, and 0.2 mM NADH in a final volume of 2 ml. The reaction was started by the addition of 20 pmol nd V/A-ATPase to 2 ml of the assay mixture, and the rate of ATP hydrolysis was monitored as the rate of oxidation of NADH was determined by the absorbance decrease at 340 nm. Cryo-EM imaging of Tth V/A-ATPase Sample vitrification was performed using a semi-automated vitrification device (Vitrobot, FEI). For nd -V/A-ATPase that underwent nucleotide removal, hereafter referred to as nucfree nd -V/A-ATPase, 2.4 μl of sample solution at a concentration of 3 mg/ml (2 μM) was applied to glow discharged Quantifoil R1.2/1.3 molybdenum grid discharged by Ion Bombarder (Vacuum Device) for 1 min. The grid was then automatically blotted once from both sides with filter paper for 6 s blot time. The grid was then plunged into liquid ethane with no delay time. The reaction basal buffer (RB buffer) containing 50 mM Tris-Cl, pH 8.0, 100 mM KCl, and 2 mM MgCl 2 was used for different reaction conditions. For saturated ATP or ATP waiting condition, 4 µM of nucfree nd -V/A-ATPase was mixed with the same volume of ×2 RB buffer containing 10 mM PEP, 200 μg/ml of PK, 12 mM, or 100 µM of ATP-Mg. Then the mixtures were incubated for 120 or 300 s at 25 °C, followed by blotting and vitrification, respectively. For the ATPγS saturated condition, 4 µM of nucfree nd -V/A-ATPase was mixed with the same volume of ×2 RB buffer containing 8 mM ATPγS-Mg, then incubated for 300 s at 25 °C, followed by the blotting and vitrification. With the exception of the saturated ATPγS condition, cryo-EM imaging was performed with a Titan Krios (FEI/Thermo Fisher) operating at 300 kV acceleration voltage and equipped with a direct K3 (Gatan) electron detector in electron counting mode (CDS). Data collection were carried out using SerialEM software [36] at a calibrated magnification of 0.88 Å pixel −1 (×81,000) and a total dose of 50.0 e − Å −2 (or 1.0 e − Å −2 per frame) (where e − specifies electrons) with a total 5 s exposure time. The defocus range was −0.8 to −2.0 μm. The data were collected as 50 movie frames. For the saturated ATPγS condition, Cryo-EM movie collection was performed with a CRYOARM 300 (JEOL) operating at 300 keV accelerating voltage and equipped with a K3 (Gatan) direct electron detector, in electron counting mode (CDS) using the data collection software serialEM. The pixel size was 1.1 Å/pix (×60,000) and a total dose of 50.0 e − Å −2 (1.0 e − Å −2 per frame) with a total 3.0 s exposure time (50 frames) with a defocus range of −1.0 to −3.5 μm. Image processing Image processing steps for each reaction condition are summarized in Supplementary Fig. 3a–d . Image analysis software, Relion 3.1 and Cryosparc 3.2, were used [37] , [38] . CTFFIND 4.1 and MotionCor2 were used for CTF estimation and movie correction in Relion [39] , [40] . Topaz software was used for machine-learning-based particle picking [41] . We started with 15,317 movies for the nucleotide-free enzyme (nucfree nd -V/A-ATPase), 13,164 movies for saturated ATP condition, 15,711 movies for saturated ATP condition, and 17,522 movies for ATPγS condition. The software used in the steps is indicated in the figure. Autopicking based on template matching or based on Topaz machine-learning resulted in 4,354,341 particles for the nucfree nd -V/A-ATPase, 2,300,834 particles for the ATP saturated condition, 1,671,397 particles for the ATP waiting condition, and 4,677.284 particles for the ATPγS waiting condition. Particles were extracted at 5x the physical pixel size from the movie-corrected micrographs and selected using 2D or 3D classification (nucfree nd-V/A-ATPase; 132,904 particles, saturated ATP; 188,673 particles, ATP waiting; 186,928 particles, ATPγS; 197,960 particles). The selected particles were extracted at full pixel size and subjected to 3D auto-refinement refollowed by CTF refinement by Bayesian polishing. Another round of 3D auto-refine, CTF refinement, and a final round of masked auto-refinement gave holo -V/A-ATPase maps at between 2.7 and 6.3 Å resolution. The membrane domain was visible but not particularly clear compared to the hydrophilic V 1 domain in a holo- enzyme map. This seemed to be due to the structural flexibility between the membrane domain and V 1 in the holo -enzyme. Focused refinement with signal subtraction targeting the V 1 EG region improved the map quality of the V 1 EG region (Supplementary Fig. 3a–d ). The refinements provided the density maps for V 1 EG under each condition at 2.8–4.1 Å resolution. After the focused refinement, masked classification on A open and B semi subunits was carried out to classify the conformational differences. The resolution was based on the gold standard Fourier shell correlation = 0.142 criterion. Model building and refinement To generate the atomic model for the V 1 EG region of V/A-ATPase, the individual subunits of the V 1 EG model from the previous structure of V/A-ATPase (PDBID: 6QUM) were fitted into the density map as rigid bodies [25] with particular focus on the N terminal region of EG stalk (E; 1–77 aa., G; 2–33 aa). The rough initial model was refined against the map with Phenix suite phenix.real_space_refine program [42] . The initial model was extensively manually corrected residue by residue in COOT [42] in terms of side-chain conformations. Peripheral stalks were removed due to low resolution in this region. The corrected model was again refined by the phenix.real_space_refine program with secondary structure and Ramachandran restraints, then the resulting model was manually checked by COOT. This iterative process was performed for several rounds to correct remaining errors until the model was in good agreement with geometry, as reflected by the MolProbity score of 1.08–1.74 and EMRinger score of 1.59–3.94 [43] , [44] . For model validation against over-fitting, the built models were used for calculation of FSC curves against both half maps, and compared with the FSC of the final model against the final density map used for model building by phenix.refine program. The statistics of the obtained maps and the atomic model were summarized in Supplementary Tables 4 – 11 . RMSD values between the atomic models were calculated using UCSF chimera [45] . 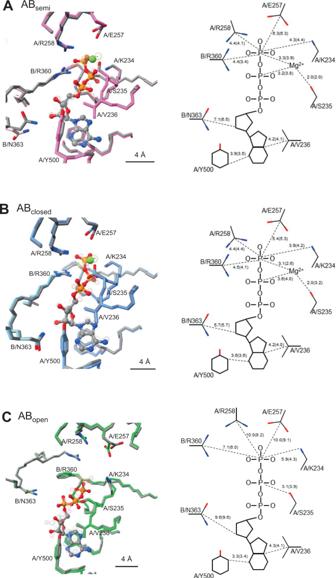Fig. 5: Coordination of nucleotides in the binding sites of V3nucand Vprehyd. Left panels;Comparison of the three nucleotide-binding sites (ABopen(A), ABsemi(B), and ABclosed(C)) of state1–1 of V3nucshown with colored (green, blue, and pink) atoms and bonds, and main chain, and state1–1 of Vprehydshown with gray atoms, bonds and main chain.Right panels;schematic representations of the coordination of the ATP group in the three binding sites of V3nucand Vprehydin parentheses. The distances between the atoms are shown in dotted lines. All distances are in Å. All the figures were rendered using UCSF chimeraX [46] . 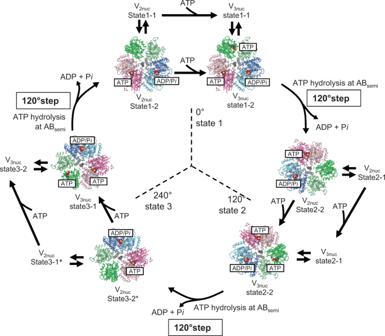Fig. 6: Chemo-Mechanical cycle of V/A-ATPase driven by ATP hydrolysis. The structures of V/A-ATPase viewed from the cytosolic side are shown as ribbon models. The coiled-coil of the DF subunits is shown in gray. The bound ATP molecules are highlighted in sphere representations. State1–1 and 1–2 of V2nucare in equilibrium and are fluctuating. These structures transit to state1–1 and 1–2 of V3nucby ATP binding to ABopen, without a 120° rotation step of the DF rotor. V3nucin state1–1 and state1–2 are also in equilibrium. ATP hydrolysis at ABsemiand zipper motion at ABopenoccur simultaneously. This triggers the transition of V3nucin state1–2 to V2nucstate2–2 together with the 120° rotation step and simultaneous release of ADP andPi. State2 of V2nucreturns to state1 via state3 of V2nucby the same process. Asterisks indicate the structures which were not identified in this study. 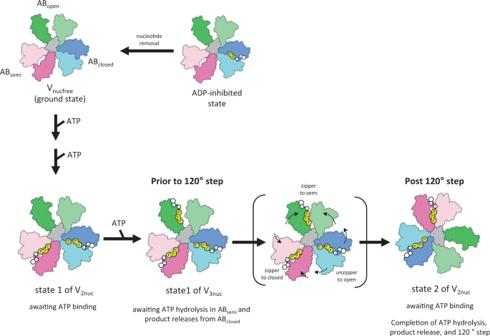Fig. 7: The rotary mechanism of V/A-ATPase powered by ATP hydrolysis. The schematic models of ABopen, ABsemi, and ABclosedare shown in green, pink, and blue, respectively. The coiled-coil region of the D subunit in contact with A3B3is shown in gray. In the ADP inhibited state, the entrapped ADP in ABclosedhampers the structural transition of ABopento ABsemiby binding of ATP to ABopen. The Vnucfreein the ground state is activated by the binding of ATP to the catalytic sites. In V2nucawaiting ATP binding, binding of ATP to ABopendoes not induce the 120° rotation step. In V3nuc, both zipper motion of ABopenand ATP hydrolysis in ABsemiinduce unzipper motion of ABclosedaccompanying the release of ADP andPi. The catalytic events in the three AB dimers occur simultaneously with the 120˚ step of the DF shaft, resulting in the structural transition of state1 of V3nucto state2 of V2nuc. Reporting summary Further information on research design is available in the Nature Research Reporting Summary linked to this article.